The NLRP3 inflammasome is critically involved in the development of bronchopulmonary dysplasia The pathogenesis of bronchopulmonary dysplasia (BPD), a devastating lung disease in preterm infants, includes inflammation, the mechanisms of which are not fully characterized. Here we report that the activation of the NLRP3 inflammasome is associated with the development of BPD. Hyperoxia-exposed neonatal mice have increased caspase-1 activation, IL1β and inflammation, and decreased alveolarization. Nlrp3 −/− mice have no caspase-1 activity, no IL1β, no inflammatory response and undergo normal alveolarization. Treatment of hyperoxia-exposed mice with either IL1 receptor antagonist to block IL1β or glyburide to block the Nlrp3 inflammasome results in decreased inflammation and increased alveolarization. Ventilated preterm baboons show activation of the NLRP3 inflammasome with increased IL1β:IL1ra ratio. The IL1β:IL1ra ratio in tracheal aspirates from preterm infants with respiratory failure is predictive of the development of BPD. We conclude that early activation of the NLRP3 inflammasome is a key mechanism in the development of BPD, and represents a novel therapeutic target for BPD. Bronchopulmonary dysplasia (BPD), a common pulmonary complication seen in preterm infants, has a multifactorial pathogenesis [1] . An inflammatory response with elaboration of growth factors and cytokines is associated with the development of BPD [2] , [3] . Pathogen or endogenous danger signals are recognized by specific pattern recognition receptors that promote a nonspecific, yet robust response to mobilize inflammatory cells [4] . These include Toll-like receptors (TLRs), the activation of which results in the transcription of cytokines, especially pro-IL1β, as well as a family of exclusively intracellular proteins called NOD-like receptors (NLRs) [5] . One such NLR, NACHT, LRR and PYD domains-containing protein 3 (NALP3), encoded by the NLR family, pyrin domain containing 3 ( NLRP3 ) gene, forms a protein complex with the adaptor molecule apoptosis-associated Speck-like protein containing a CARD (ASC) and procaspase-1 to form the NLRP3 inflammasome [6] . Formation of this complex results in the processing of procaspase-1 to an active 20 kDa fragment that enzymatically cleaves pro-IL1β to mature IL1β [6] . Studies suggest that IL1β exists in balance with its receptor antagonist IL1ra, and an increased IL1β:IL1ra ratio initiates inflammation that has been implicated in human diseases [7] , [8] , [9] . Recently, the Nlrp3 inflammasome was implicated in an adult mouse model of hyperoxia-induced acute lung injury [10] . However, whether the NLRP3 inflammasome is operative in BPD, either in animal models of the disease or in infants destined to develop BPD, is unknown. In this study, we found that the Nlrp3 inflammasome is activated in neonatal mice exposed to 85% oxygen (O 2 ), and that it is a key mediator of the inflammation and decreased alveolarization observed in this model of BPD. Furthermore, the NLRP3 inflammasome is activated in a preterm baboon model of BPD, where ventilated baboons had an increased IL1β:IL1ra ratio when compared with gestational age controls. Moreover, IL1β, IL1ra and the IL1β:ILra ratio in tracheal aspirates obtained in the first 3 days after birth from human preterm infants with respiratory failure were independently predictive of adverse outcome at 36 weeks postmenstrual age (PMA). These cumulative findings reveal that the NLRP3 inflammasome is critically involved in the pathogenesis of BPD, and that it represents a novel therapeutic target for this devastating disorder of infancy. In particular, our data defines a specific population of infants that can be targeted for therapeutic intervention in clinical trials. Nlrp3 −/− mice are protected from neonatal hyperoxia To determine the contribution of Nlrp3 to the development of BPD, we examined wild-type (WT) and Nlrp3 −/− mice in a neonatal model of hyperoxia-induced BPD. Compared with controls, exposure to 85% O 2 resulted in a 40-fold increase in whole lung IL1β mRNA on PN10 in both WT and Nlrp3 −/− (PN10, Fig. 1a ), suggesting that pro-IL1β expression is similarly upregulated in both groups. However, whereas WT mice exposed to 85% O 2 had a 10-fold increase in mature IL1β protein in bronchoalveolar lavage (BAL) by PN15, Nlrp3 −/− mice had undetectable BAL IL1β protein ( Fig. 1b ). Caspase-1 activity in whole-lung tissue was increased twofold in WT mice in 85% O 2 , but was undetectable in Nlrp3 −/− mice ( Fig. 1c ), and lung p20 caspase-1 was increased in WT and was not detectable in Nlrp3 −/− mice exposed to 85% O 2 ( Fig. 1d ). Similarly, Nlrp3 −/− mice were unable to process pro-IL18 to mature IL18 ( Supplementary Fig. 1a and b ). These data confirmed that the Nlrp3 −/− mice were able to generate pro-IL1β and pro-IL18, but not process them to mature IL1β and IL18. 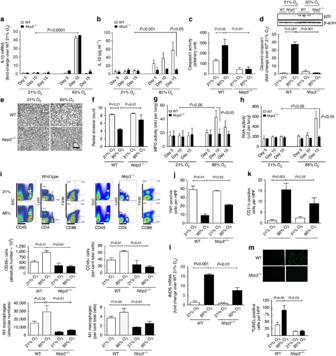Figure 1:Nlrp3−/−mice are protected from neonatal hyperoxia-induced inflammation and decreased alveolarization. All data are expressed as mean±s.e.m. withn=6–12 animals per group for each experiment. (a) Mice exposed to 85% O2had a 45-fold increase in IL1β mRNA. (b) In BAL, WT mice exposed to hyperoxia had increased mature IL1β protein, whereasNlrp3−/−mice had no detectable mature IL1β. (c) Lung caspase-1 activity was increased threefold in WT mice exposed to 85% O2, but was undetectable inNlrp3−/−mice. (d) Hyperoxia-exposed WT mice had a 35-fold increase in p20-cleaved caspase-1. Animals in 21% O2andNlrp3−/−mice exposed to 85% O2had no detectable p20. (e) On PN15, WT lungs obtained had decreased secondary septation, whereasNlrp3−/−mice had normal alveolarization (Scale bar, 400 μm). (f) WT mice exposed to 85% O2had decreased radial alveolar count (RAC), whereasNlrp3−/−mice had normal RAC. (g) MPO activity of lavage cell pellets was increased maximally on day 10 in WT animals exposed to 85% O2, but was unchanged in WT mice kept in 21% O2and inNlrp3−/−mice in either condition. (h) NAG activity of lavage cell pellets was increased on day 15 in WT animals exposed to 85% O2, but was unchanged in WT mice kept in 21% O2and inNlrp3−/−mice under either condition. (i) Single-cell preparations of lungs from WT orNlrp3−/−mice were subjected to flow cytometry to identify total white cells (CD45), neutrophils (Ly6G), lymphocytes (CD4), macrophages (F4/80) and M1 macrophages (CD86). WT mice, but notNlrp3−/−mice, exposed to hyperoxia had increased absolute numbers and per cent total CD45+ cells and M1 macrophages. (j) By immunofluorescence, WT mice had high expression of YM1 that decreased with exposure to 85% O2. This decrease was significantly less inNlrp3−/−mice in 85% O2. (k) By immunofluorescence, expression of CD11c was low to undetectable in WT mice and increased with 85% O2. This increase was blunted inNlrp3−/−mice in 85% O2. (l) Steady-state mRNA content of iNOS confirmed the CD11c findings. (m) WT mice exposed to 85% O2had increased TUNEL-positive cells, whereasNlrp3−/−had no evidence of apoptosis in any condition. Figure 1: Nlrp3 −/− mice are protected from neonatal hyperoxia-induced inflammation and decreased alveolarization. All data are expressed as mean±s.e.m. with n =6–12 animals per group for each experiment. ( a ) Mice exposed to 85% O 2 had a 45-fold increase in IL1β mRNA. ( b ) In BAL, WT mice exposed to hyperoxia had increased mature IL1β protein, whereas Nlrp3 −/− mice had no detectable mature IL1β. ( c ) Lung caspase-1 activity was increased threefold in WT mice exposed to 85% O 2 , but was undetectable in Nlrp3 −/− mice. ( d ) Hyperoxia-exposed WT mice had a 35-fold increase in p20-cleaved caspase-1. Animals in 21% O 2 and Nlrp3 −/− mice exposed to 85% O 2 had no detectable p20. ( e ) On PN15, WT lungs obtained had decreased secondary septation, whereas Nlrp3 −/− mice had normal alveolarization (Scale bar, 400 μm). ( f ) WT mice exposed to 85% O 2 had decreased radial alveolar count (RAC), whereas Nlrp3 −/− mice had normal RAC. ( g ) MPO activity of lavage cell pellets was increased maximally on day 10 in WT animals exposed to 85% O 2 , but was unchanged in WT mice kept in 21% O 2 and in Nlrp3 −/− mice in either condition. ( h ) NAG activity of lavage cell pellets was increased on day 15 in WT animals exposed to 85% O 2 , but was unchanged in WT mice kept in 21% O 2 and in Nlrp3 −/− mice under either condition. ( i ) Single-cell preparations of lungs from WT or Nlrp3 −/− mice were subjected to flow cytometry to identify total white cells (CD45), neutrophils (Ly6G), lymphocytes (CD4), macrophages (F4/80) and M1 macrophages (CD86). WT mice, but not Nlrp3 −/− mice, exposed to hyperoxia had increased absolute numbers and per cent total CD45+ cells and M1 macrophages. ( j ) By immunofluorescence, WT mice had high expression of YM1 that decreased with exposure to 85% O 2 . This decrease was significantly less in Nlrp3 −/− mice in 85% O 2 . ( k ) By immunofluorescence, expression of CD11c was low to undetectable in WT mice and increased with 85% O 2 . This increase was blunted in Nlrp3 −/− mice in 85% O 2 . ( l ) Steady-state mRNA content of iNOS confirmed the CD11c findings. ( m ) WT mice exposed to 85% O 2 had increased TUNEL-positive cells, whereas Nlrp3 −/− had no evidence of apoptosis in any condition. Full size image The lungs of WT and Nlrp3 −/− mice exposed to either 21% or 85% O 2 were examined at PN5, PN10 and PN15. Distal lung histology on PN15 in WT mice exposed to 85% O 2 showed simplification of the distal lung architecture with larger saccular structures ( Fig. 1e ). Morphometric analysis at PN15 using radial alveolar count (RAC) demonstrated decreased alveolarization in WT mice ( Fig. 1f ). In contrast, Nlrp3 −/− mice had a normal, complex distal lung architecture with well-formed alveoli and a normal RAC ( Fig. 1e,f ). We next determined the influx of neutrophils and macrophages into the lung by measuring specific enzyme activities in cell pellets obtained after BAL, namely myeloperoxidase (MPO) and N-acetyl glucosaminidase (NAG) activities, respectively. Of note, NAG activity was not increased in resident alveolar macrophages either at baseline or after TLR2 or 4 stimulation, whereas bone marrow-derived macrophages (BMDMs) had increased NAG activity, both at baseline and after TLR stimulation ( Supplementary Fig. 1c ). WT mice in 85% O 2 had a maximal increase in MPO activity on PN10 ( Fig. 1g ), whereas NAG activity was increased at PN15 ( Fig. 1h ). These increases were not seen in Nlrp3 −/− mice ( Fig. 1g,h ). We next determined the composition of inflammatory cells using flow cytometry of whole-lung single-cell preparations from WT and Nlrp3 −/− mice ( Fig. 1i ). In WT mice, exposure to 85% O 2 resulted in a twofold increase in absolute numbers of CD45 + cells (accounting for 50% of the total number of cells), and a specific increase (twofold in absolute numbers and 25% of total cells) in M1 macrophages (Ly6G − , CD4F4/80 + , CD86 + ; Fig. 1i ). In contrast, Nlrp3 −/− mice exposed to 85% O 2 failed to show these increases in both CD45 + cells and M1 macrophages ( Fig. 1i ). We also determined the phenotype of macrophages by staining tissue sections for specific markers. Based on the high expression of YM1 and low expression of CD11c, WT animals in 21% O 2 had a predominantly M2 or alternatively activated macrophages ( Fig. 1j,k ). Exposure of WT mice to 85% O 2 resulted in decreased numbers of YM1-positive cells per high power field (HPF) and increased numbers of CD11c-positive cells per HPF ( Fig. 1j,k ), suggesting a switch to the M1 or classically activated phenotype. The mRNA of an alternate M1 marker, inducible nitric oxide synthase (iNOS) was also increased in WT mice exposed to 85% O 2 ( Fig. 1l ). Nlrp3 −/− mice exposed to 85% O 2 were protected from this phenotypic switch and had higher expression of YM1 and lower expression of CD11c and iNOS as compared with WT mice exposed to 85% O 2 ( Fig. 1j–l ). We confirmed these changes in M2 to M1 macrophage phenotypes by examining the expression of active transforming growth factor-β1 (TGFβ1), tumour necrosis factor-α (TNFα) and G-CSF, all of which were increased in WT, but not in Nlrp3 −/− mice exposed to 85% O 2 ( Supplementary Fig. 1d,e and f ). Using Terminal transferase dUTP nick-end labelling (TUNEL) staining, we also determined apoptosis in the lung. Exposure of WT mice to 85% O 2 was associated with an increased number of TUNEL-positive cells, and this was completely abrogated in Nlrp3 −/− mice ( Fig. 1m ). Collectively, these data demonstrated that Nlrp3 is a critical component of the neonatal mouse response to hyperoxia and regulates inflammation and subsequent effects on alveolarization. Pharmacologic inhibition of IL1β or the Nlrp3 inflammasome Given that genetic deletion of Nlrp3 was associated with complete protection from hyperoxia-induced changes in lung inflammation and alveolar architecture, we next sought to block this pathway pharmacologically in WT mice using either recombinant IL1ra (which blocks IL1β interaction with its receptor [8] ), or glyburide (which prevents the formation of the Nlrp3 inflammasome [11] ). Caspase-1 activity was similarly increased in both vehicle- and IL1ra-treated mice, suggesting that the formation of the Nlrp3 inflammasome was intact in both these conditions ( Fig. 2a ). This was confirmed by western blot for the p20 active fragment of caspase-1, which was present in both vehicle- and IL1ra-treated lungs of hyperoxia-exposed mice ( Fig. 2b ). Expression of IL1β mRNA, as a surrogate for pro-IL1β, was increased equally in both vehicle- and IL1ra-treated groups, though the IL1ra-treated group had a lower IL1β mRNA than controls ( Supplementary Fig. 2a ), suggesting a positive feedback loop for the stimulation of IL1β transcription. Similarly, while mature IL1β was increased in hyperoxia-exposed mice, there was less mature IL1β protein in IL1ra-treated mice compared with controls ( Supplementary Fig. 2b ). Compared with vehicle-treated mice, IL1ra-treated mice were protected from decreased alveolarization seen with exposure to 85% O 2 ( Fig. 2c,d ). As seen with Nlrp3 −/− mice in hyperoxia, both increased MPO and NAG activities were abrogated with IL1ra treatment ( Fig. 2e,f ), suggesting that blockade of IL1β alone was sufficient to block the inflammatory response to injury. As seen with Nlrp3 −/− mice, IL1ra treatment resulted in decreased apoptosis, as well as decreased TGFβ1 and TNFα expression ( Supplementary Fig. 2c,d and e ). 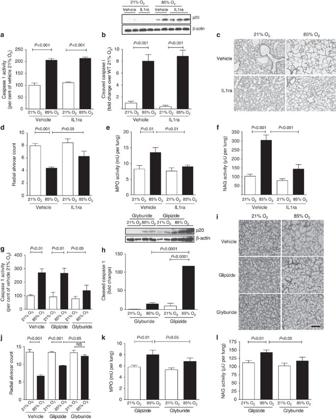Figure 2: WT mice exposed to 85% O2are protected when treated with either recombinant IL1ra to block IL1β receptor or glyburide to block formation of the Nlrp3 inflammasome. All data are presented as mean±s.e.m. withn=6–12 animals per group. (a) The lungs of WT mice exposed to 85% O2had equally increased caspase-1 activity in both vehicle and IL1ra-treated mice. (b) All mice in 85% O2, both vehicle- and IL1ra-treated, showed an eightfold increase in p20-cleaved caspase-1. None of the 21% O2animals had the p20-cleaved protein. (c) Vehicle-treated mice exposed to 85% O2had decreased secondary septation. Mice exposed to 85% O2and treated with IL1ra had improved alveolarization as compared with vehicle-treated controls. (d) Exposure of WT mice to 85% O2resulted in decreased RAC. Treatment of hyperoxia-exposed mice with IL1ra significantly improved RAC. (e) MPO activity of lavage cell pellets was increased in vehicle-treated, 85% O2-exposed mice and this was abrogated with treatment with IL1ra. (f) The NAG activity of lavage cell pellets was increased in vehicle-treated, 85% O2-exposed mice, and treatment with IL1ra prevented this increase. (g) WT mice in 85% O2had increased caspase-1 activity either with vehicle or glipizide treatment. Mice in 85% O2treated with glyburide caspase-1 activity similar to 21% O2animals. (h) Only 85% O2-exposed animals given glipizide, and not those treated with glyburide, had increased p20-cleaved caspase-1. (i) On PN15, WT lungs exposed to 85% O2with either vehicle or glipizide had decreased secondary septation, whereas 85% O2-exposed mice treated with glyburide had normal alveolarization (Scale bar, 400 μm). (j) Exposure to 85% O2and treatment with either vehicle or glipizide results in decreased RAC. Treatment with glyburide, normalized RAC. (k) MPO activity was increased in BAL cell pellets from 85% O2-exposed mice treated with glipizide, whereas mice treated with glyburide had no increase in MPO. (l) The NAG activity of BAL cell pellets was increased in glipizide-treated, 85% O2-exposed mice. However, treatment of hyperoxia-exposed mice with glyburide prevented this increase in NAG activity. Figure 2: WT mice exposed to 85% O 2 are protected when treated with either recombinant IL1ra to block IL1β receptor or glyburide to block formation of the Nlrp3 inflammasome. All data are presented as mean±s.e.m. with n =6–12 animals per group. ( a ) The lungs of WT mice exposed to 85% O 2 had equally increased caspase-1 activity in both vehicle and IL1ra-treated mice. ( b ) All mice in 85% O 2 , both vehicle- and IL1ra-treated, showed an eightfold increase in p20-cleaved caspase-1. None of the 21% O 2 animals had the p20-cleaved protein. ( c ) Vehicle-treated mice exposed to 85% O 2 had decreased secondary septation. Mice exposed to 85% O 2 and treated with IL1ra had improved alveolarization as compared with vehicle-treated controls. ( d ) Exposure of WT mice to 85% O 2 resulted in decreased RAC. Treatment of hyperoxia-exposed mice with IL1ra significantly improved RAC. ( e ) MPO activity of lavage cell pellets was increased in vehicle-treated, 85% O 2 -exposed mice and this was abrogated with treatment with IL1ra. ( f ) The NAG activity of lavage cell pellets was increased in vehicle-treated, 85% O 2 -exposed mice, and treatment with IL1ra prevented this increase. ( g ) WT mice in 85% O 2 had increased caspase-1 activity either with vehicle or glipizide treatment. Mice in 85% O 2 treated with glyburide caspase-1 activity similar to 21% O 2 animals. ( h ) Only 85% O 2 -exposed animals given glipizide, and not those treated with glyburide, had increased p20-cleaved caspase-1. ( i ) On PN15, WT lungs exposed to 85% O 2 with either vehicle or glipizide had decreased secondary septation, whereas 85% O 2 -exposed mice treated with glyburide had normal alveolarization (Scale bar, 400 μm). ( j ) Exposure to 85% O 2 and treatment with either vehicle or glipizide results in decreased RAC. Treatment with glyburide, normalized RAC. ( k ) MPO activity was increased in BAL cell pellets from 85% O 2 -exposed mice treated with glipizide, whereas mice treated with glyburide had no increase in MPO. ( l ) The NAG activity of BAL cell pellets was increased in glipizide-treated, 85% O 2 -exposed mice. However, treatment of hyperoxia-exposed mice with glyburide prevented this increase in NAG activity. Full size image Since IL1ra treatment did not disrupt the formation of the Nlrp3 inflammasome, we next examined the effects of glyburide, which interferes with the formation of the Nlrp3-Asc-caspase-1 complex [11] . Since glipizide is also an anti-diabetic drug in the same class as glyburide, but has no effect on the Nlrp3 complex, we used this, in addition to vehicle alone, as a control. With hyperoxia exposure, caspase-1 activity was increased in mice treated with either vehicle or glipizide. However, mice treated with glyburide had a lower caspase-1 activity ( Fig. 2g ). Western blot showed increased expression of the cleaved p20-active caspase-1 in glipizide-treated, hyperoxia-exposed mice. This response was completely inhibited in glyburide-treated mice suggesting that the Nlrp3 inflammasome was blocked ( Fig. 2h ). Whereas the increase in IL1β mRNA with hyperoxia was unaffected by any treatment, BAL IL1β protein was increased with hyperoxia in glipizide-treated mice, but not in glyburide-treated mice ( Supplementary Fig. 2f and g ). Exposure to hyperoxia in mice treated with vehicle or glipizide was associated with decreased alveolarization, whereas treatment with glyburide resulted in normal alveolarization ( Fig. 2i,j ). In addition, treatment with glyburide also abrogated neutrophil and macrophage influx as seen by decreased MPO and NAG activities as compared with glipizide-treated controls ( Fig. 2k,l ). Glyburide treatment was also associated with complete abrogation of apoptosis due to hyperoxia exposure ( Supplementary Fig. 2h ). Furthermore, active TGFβ1 and TNFα expression were increased in glipizide-treated mice, but not in glyburide-treated mice exposed to hyperoxia ( Supplementary Fig. 2i and j ). Collectively, these data suggest that activation of the Nlrp3 inflammasome is vital to the development of inflammation and the inhibition of secondary septation in hyperoxia-injured mice, and that the administration of pharmacologic agents currently in human use, namely IL1ra and glyburide, abrogate Nlrp3 inflammasome formation and its consequences to ameliorate the development of the BPD phenotype in this model. The NLRP3 inflammasome in a primate model of BPD To determine the normal ontogeny of IL1β and IL1ra in primate lung during the third trimester of pregnancy, we first obtained samples from baboons at various times in gestation. Term gestation in the baboon is 185 days. Animals were sacrificed and tracheal fluid was obtained at the time of caesarian delivery. IL1β protein, normalized to the Secretory Component of IgA (SCIgA), was low throughout pregnancy except in animals that were harvested at term after spontaneous labour ( Supplementary Fig. 3a ). Interestingly, IL1ra was highest at earlier points in gestation, decreased until 175d, and increased again in animals at term after spontaneous labour ( Supplementary Fig. 3b ). The IL1β:IL1ra ratio therefore steadily increased from 125 to 185d suggesting a gradual increase in the inflammatory potential of the lung during gestation ( Supplementary Fig. 3c ). Next, preterm baboons were delivered at 70% of gestation (125 days; ∼ 28 weeks equivalent in the human) and ventilated using standard neonatal protocols for ventilation and oxygenation for 14 days (125d+14d pro re nata (PRN)). Samples from these animals were compared with those obtained from fetal baboons harvested at either 125d or 140d as gestational age controls. The 140d gestational age control animals are at the same post-conceptual age as the 125d+14d PRN, but the last 2 weeks took place in utero . Preterm birth, ventilation and exposure to oxygen were associated with a 60-fold increase in IL1β mRNA as compared with either gestational age control ( Fig. 3a ). Caspase-1 activity was twofold higher in ventilated preterm baboons as compared with either control ( Fig. 3b ), and the content of p20 caspase-1 was higher in ventilated animals as compared with gestational controls ( Fig. 3c ). IL1β protein, normalized to SCIgA, was threefold higher in ventilated animals versus gestational controls ( Fig. 3d ), and IL1ra, also normalized to SCIgA, did not decrease as noted between 125d and 140d gestational age controls ( Fig. 3e ). The IL1β:IL1ra ratio was, therefore, significantly increased in the preterm birth with ventilation and oxygen exposure group than either gestational age control suggesting an activation of the NLRP3 inflammasome ( Fig. 3f ). Of note, the baboon model of BPD has previously been shown to develop decreased alveolarization [12] , [13] . 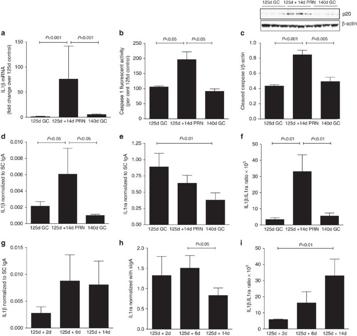Figure 3: Increased IL1β, IL1ra and IL1β:IL1ra ratio in a non-human primate model of BPD. All data are expressed as mean±s.e.m. withn=6–8 animals per group for each experiment. Preterm baboon tracheal aspirates or lung tissue obtained from 125-day gestation animals ventilated with appropriate ventilation and oxygenation for 14 days (125d+14d PRN), and either at 125 or 140 days gestation animals as controls (125d GC; 140d GC) were examined as described in Methods section. (a) IL1β mRNA was elevated 60-fold in 125-day preterm baboons ventilated for 14 days as compared with either 125- or 140-day gestational age controls. (b). Caspase-1 activity was elevated twofold in the lungs of ventilated preterm baboons as compared with the gestational age controls. (c) Cleaved p20 caspase-1 was increased twofold in ventilated preterm baboons as compared with gestational age controls. (d–f) Tracheal aspirate concentrations of IL1β and IL1ra normalized to the Secretory Component of IgA (SCIgA), and the IL1β:IL1ra ratio in the preterm baboon model. (d) BAL IL1β/SCIgA was increased threefold in ventilated preterm baboons as compared with 125- and 140-day gestational controls. (e) BAL IL1ra/SCIgA decreased from 125 to 140 days in gestational age controls. Ventilated preterm baboons had IL1ra/SCIgA levels intermediate between the two gestational ages. (f) The ratio of IL1β to IL1ra in the BAL was increased eightfold in ventilated preterm baboons as compared with 125- and 140-day gestational age controls. (g–i) Changes in IL1β/SCIgA, IL1ra/SCIgA and IL1β:IL1ra ratio were determined in tracheal aspirate samples obtained on days 2, 6 and 14 after birth. (g) Although there was a trend to increase from day 2 to day 6, there were no significant differences in IL1β/SCIgA after birth. (h) IL1ra/SCIgA decreased significantly between day 6 and day 14 after birth. (i) The ratio of IL1β to IL1ra steadily increased after birth such that it was significantly elevated by day 14 after birth. Figure 3: Increased IL1β, IL1ra and IL1β:IL1ra ratio in a non-human primate model of BPD. All data are expressed as mean±s.e.m. with n =6–8 animals per group for each experiment. Preterm baboon tracheal aspirates or lung tissue obtained from 125-day gestation animals ventilated with appropriate ventilation and oxygenation for 14 days (125d+14d PRN), and either at 125 or 140 days gestation animals as controls (125d GC; 140d GC) were examined as described in Methods section. ( a ) IL1β mRNA was elevated 60-fold in 125-day preterm baboons ventilated for 14 days as compared with either 125- or 140-day gestational age controls. ( b ). Caspase-1 activity was elevated twofold in the lungs of ventilated preterm baboons as compared with the gestational age controls. ( c ) Cleaved p20 caspase-1 was increased twofold in ventilated preterm baboons as compared with gestational age controls. ( d – f ) Tracheal aspirate concentrations of IL1β and IL1ra normalized to the Secretory Component of IgA (SCIgA), and the IL1β:IL1ra ratio in the preterm baboon model. ( d ) BAL IL1β/SCIgA was increased threefold in ventilated preterm baboons as compared with 125- and 140-day gestational controls. ( e ) BAL IL1ra/SCIgA decreased from 125 to 140 days in gestational age controls. Ventilated preterm baboons had IL1ra/SCIgA levels intermediate between the two gestational ages. ( f ) The ratio of IL1β to IL1ra in the BAL was increased eightfold in ventilated preterm baboons as compared with 125- and 140-day gestational age controls. ( g – i ) Changes in IL1β/SCIgA, IL1ra/SCIgA and IL1β:IL1ra ratio were determined in tracheal aspirate samples obtained on days 2, 6 and 14 after birth. ( g ) Although there was a trend to increase from day 2 to day 6, there were no significant differences in IL1β/SCIgA after birth. ( h ) IL1ra/SCIgA decreased significantly between day 6 and day 14 after birth. ( i ) The ratio of IL1β to IL1ra steadily increased after birth such that it was significantly elevated by day 14 after birth. Full size image To determine the changes after birth, tracheal aspirate samples were obtained from ventilated preterm baboons on days 2, 6 and 14 after birth. Compared with samples obtained on day 2, the IL1β:SCIgA ratio tended to be increased by day 6 and was sustained until 14 days of age, though this did not reach significance ( Fig. 3g ). The IL1ra:SCIgA ratio decreased between days 6 and 14 after birth ( Fig. 3h ). As a result, the IL1β:IL1ra ratio progressively increased from day 2 to day 14 when it was significantly elevated compared with the day 2 samples ( Fig. 3i ). These data suggest that the IL1β:IL1ra ratio is not elevated at birth and increases after exposure to preterm birth, ventilation and oxygen in the baboon model of BPD. Tracheal aspirate IL1β and IL1ra in preterm infants Preterm infants who develop respiratory failure requiring mechanical ventilation and exposure to increased oxygen concentrations are at risk of developing BPD. Indeed, the incidence of BPD is greater with decreasing gestation [1] . Although a number of clinical prediction models have been developed, most are poor in predicting BPD and do not address the pathogenesis of the disease [14] . To determine whether IL1β and/or IL1ra are biomarkers that could independently predict death or BPD in these infants, we conducted a prospective cohort study of 48 neonates born between 24 0/7th to 31 6/7th weeks gestation that had respiratory failure requiring intubation and ventilation. Infants with proven sepsis as evidenced by a positive blood culture, perinatal asphyxia or major congenital anomalies were excluded from the study. BPD was defined as the physiologic need for supplemental oxygen at 36 weeks PMA. Because death is a competing outcome, death or BPD was used as a primary outcome for this study. Table 1 shows the characteristics of enroled infants ( Table 1 ). As expected, infants that developed adverse outcome were lower in gestational age and birth weight, had a higher incidence of respiratory distress syndrome, spent more days on respiratory and oxygen support, and had a longer length of hospital stay ( Table 1 ). Table 1 Characteristics of enrolled infants. Full size table Tracheal aspirate samples were obtained daily for the first 10 days, then weekly until the infant was extubated. Tracheal aspirate IL1β, IL1ra and SCIgA were determined as in the preterm baboon model. Cell pellets were obtained by light centrifugation of tracheal aspirate samples. MPO and NAG enzyme activities were measured in the cell pellets to quantify neutrophils and macrophages, respectively. Data were log transformed to achieve a normal distribution. Results were analysed in epochs of days 1–3, 4–6 and 7–10 days using the mean value for each epoch. By univariate analysis, log10IL1β, log10IL1ra and log10IL1β:IL1ra ratio in the 1–3 day epoch were all significantly higher in infants that subsequently developed adverse outcome ( Fig. 4a–c ). NAG activity, as a measure of macrophage content, was elevated in the 7–10 day epoch in the group that developed adverse outcome ( Fig. 4d ). Since gestational age is a confounder for the development of BPD, we determined whether these biomarkers were related to gestational age. Using Pearson’s correlations, log10IL1β, log10IL1ra and log10IL1β:IL1ra ratio in the 1–3 day epoch were each inversely correlated with gestational age, having a higher value at lower gestational age ( Supplementary Fig. 4a,b and c ). Using logistic regression analysis, each of the three parameters, log10IL1β, log10IL1ra and log10IL1β:IL1ra ratio in the 1–3 day epoch were positively associated with adverse outcome, even when controlled for the effects of gestational age ( Table 2 ). 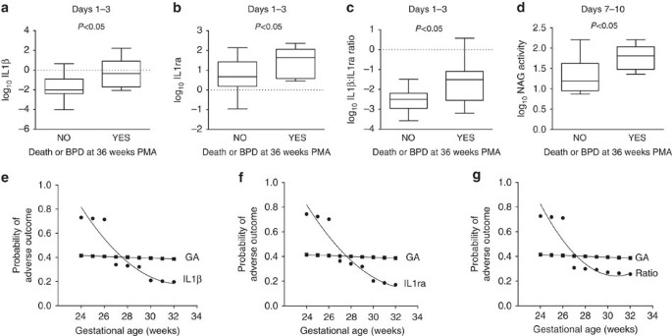Figure 4: Tracheal aspirate IL1β, IL1ra and N-acetyl glucosaminidase activity are associated with adverse outcome in preterm infants intubated for respiratory failure. (a–c) Box plots of log-transformed IL1β, IL1ra and IL1β:IL1ra ratio in tracheal aspirates obtained between days 1 and 3 segregated by adverse outcome (death or BPD at 36 weeks PMA). Each biomarker was significantly elevated between days 1 and 3 in infants that subsequently developed adverse outcome at 36 weeks PMA. (d) Box plot of log-transformed NAG activity between days 7 and 10 segregated by adverse outcome. NAG activity at 710 days was increased in those infants that developed death or BPD at 36 weeks PMA. (e–g) Comparisons of the contribution of gestational age and each of the tracheal aspirate biomarkers to the probability of adverse outcome at each gestational age. Using the 50th percentile value for each biomarker at 1–3 days, the probability of adverse outcome at each gestational age was determined and compared with the contribution of gestational age alone. Gestational age alone contributed 40% to the probability of adverse outcome at each gestational age. For infants <27 weeks gestation, each biomarker (IL1β, IL1ra and IL1β:IL1ra ratio) doubled the probability of adverse outcome above that of gestational age alone. Figure 4: Tracheal aspirate IL1β, IL1ra and N-acetyl glucosaminidase activity are associated with adverse outcome in preterm infants intubated for respiratory failure. ( a – c ) Box plots of log-transformed IL1β, IL1ra and IL1β:IL1ra ratio in tracheal aspirates obtained between days 1 and 3 segregated by adverse outcome (death or BPD at 36 weeks PMA). Each biomarker was significantly elevated between days 1 and 3 in infants that subsequently developed adverse outcome at 36 weeks PMA. ( d ) Box plot of log-transformed NAG activity between days 7 and 10 segregated by adverse outcome. NAG activity at 710 days was increased in those infants that developed death or BPD at 36 weeks PMA. ( e – g ) Comparisons of the contribution of gestational age and each of the tracheal aspirate biomarkers to the probability of adverse outcome at each gestational age. Using the 50th percentile value for each biomarker at 1–3 days, the probability of adverse outcome at each gestational age was determined and compared with the contribution of gestational age alone. Gestational age alone contributed 40% to the probability of adverse outcome at each gestational age. For infants <27 weeks gestation, each biomarker (IL1β, IL1ra and IL1β:IL1ra ratio) doubled the probability of adverse outcome above that of gestational age alone. Full size image Table 2 Logistic regression analysis of the association of biomarkers to adverse the outcome in preterm infants after controlling for gestational age. Full size table We then performed a probability analysis of adverse outcome at each gestational age as determined by the 50th percentile value of each biomarker, comparing them with the effect of gestational age alone, on the probability of adverse outcome. The contribution of gestational age to the probability of adverse outcome remained ∼ 0.4 at each gestational age examined ( Fig. 4e–g ). For infants <27 weeks gestation at birth, each of the three biomarkers examined were more predictive of adverse outcome than gestational age alone, reaching 0.75 probability of adverse outcome ( Fig. 4e–g ). Thus, infants <27 weeks gestation that exhibit at least a 50th percentile value for IL1β, IL1ra or IL1β:IL1ra ratio on day 1 to 3 of life carry the highest risk of adverse outcome, with better prediction than gestational age alone. We have explored the critical role of the NLRP3 inflammasome in the pathogenesis of BPD. Exposure to oxygen and/or ventilation, particularly in the face of premature birth, results in an increase in the activity of the NLRP3 inflammasome driving an inflammatory response. Blockade of IL1β or the Nlrp3 inflammasome results in decreased inflammation and better alveolarization, thereby ameliorating the BPD phenotype. Importantly, IL1β and its naturally occurring antagonist IL1ra are early and independent biomarkers associated with adverse outcome in premature babies, allowing the potential early identification of a subgroup of patients at particular risk that can be specifically targeted in therapeutic trials. Contrary to a recent suggestion of the lack of concordance in the responses to inflammatory stimuli between the mouse and human [15] , our findings in preterm infants with respiratory failure are fully consistent with those from murine and non-human primate models of BPD. A number of investigators have reported the association of an inflammatory influx with subsequent development of BPD in preterm infants with lung disease [2] , [16] , [17] , [18] , [19] . Elastase activity and neutrophil counts in tracheal aspirates of intubated preterm infants in the first week of life are higher in infants that subsequently develop BPD [20] . Tracheal aspirates from these infants not only have higher neutrophil counts, but also have increased concentrations of neutrophil chemoattractants such as IL8 (ref. 21 ). Neutrophil and macrophage accumulation in tracheal aspirates commences early in the first week of life and counts remain elevated in infants that develop BPD [22] , [23] . While our flow cytometry data demonstrate increased accumulation of total inflammatory cells, as well as M1 macrophages in the lungs of WT mice exposed to hyperoxia, and that these responses are completely abrogated in Nlrp3 −/− mice, it should be noted that the myeloid system in the murine lung is more diverse and complex. Becher et al. [24] , using a 38 antibody high-dimensional flow cytometry analysis identified multiple subsets of murine myeloid lineages in the lung, including more ambiguous subsets and intermediate cell types. Such a detailed study of the changes in the myeloid response to neonatal hyperoxia exposure in both WT and Nlrp3 −/− mice is warranted. Interleukin-1β (IL1β), a key initiator of inflammation, has a complex activation system and has been implicated in inflammatory disorders in humans [25] . Neonatal Onset Multisystem Inflammatory Disorders (NOMID), a collection of diseases with an imbalance in the IL1β:IL1ra ratio, are characterized by relapsing fevers and recurrent bouts of inflammation that can affect the skin, joints, bones, eyes, GI tract and the nervous system [26] . The commonest mutations in these diseases are either activating mutations of NLRP3 or inactivating mutations of IL1ra [27] . A number of inflammasomes have been described. Each consists of a sensor molecule that uses the adaptor molecule ASC to recruit and activate pro-caspase-1 (ref. 28 ). The different NLRs that make up these inflammasomes recognize specific molecules, such as bacterial peptidoglycan recognized by NLRP1 (ref. 29 ). NLRP3 senses a variety of signals including crystalline material (as in gout), peptide aggregates and bacterial toxins [29] . Our data effectively implicates NLRP3 as the principal NLR involved in the pathogenesis of BPD. With respect to BPD, elevated concentrations of IL1β in amniotic fluid [30] and postnatally [22] , [31] , [32] have been associated with the development of BPD. Indeed, in preterm infants at risk of BPD, the IL1β:IL1ra ratio is increased by days 5–7 in infants that subsequently developed BPD [9] . Furthermore, transgenic overexpression of mature IL1β in lung epithelial cells, even in the absence of hyperoxia, results in inflammation, airway remodelling and distal alveolar simplification, changes reminiscent of BPD [33] , [34] , [35] . Using this model and by crossing these mice with specific knockout mice, Bry et al. [35] have examined the downstream effects of IL1β, showing that activation of TGFβ is necessary for the BPD phenotype. While all these studies implicate IL1β and its downstream consequences, the present study is the first loss-of-function study of the Nlrp3 inflammasome in preventing oxygen-induced lung injury in neonatal mice. Our data during gestation in the baboon model show that the NLRP3 inflammasome is quiescent in utero , and increases activity with labour and birth at term gestation ( Supplementary Fig. 3 ). In addition, IL1β and IL1ra concentrations increase from day 2 to day 14 after birth in preterm baboons that are ventilated and exposed to oxygen ( Fig. 3i ). Sharma et al. [36] recently reported that NLRP3 activity in human umbilical cord blood monocytes is suppressed with a developmental lack of caspase-1 activity in infants <29 weeks gestation. Importantly, these responses matured rapidly and reached adult values in 24–29 week gestation preterm infants after birth. Collectively, these data suggest that the activation of the NLRP3 inflammasome at a time when it is normally quiescent contributes to the pathogenesis of inflammation and the development of BPD. It is likely that over-distension during mechanical ventilation as well as hyperoxia contribute to the activation of the Nlrp3 inflammasome. Indeed, mechanical stretch of macrophages in vitro and adult mouse lungs in vivo in the absence of hyperoxia exposure results in activation of Nlrp3 and production of IL1β (ref. 37 ). While thioredoxin-interacting protein has been shown to link oxidative stress to inflammasome activation [38] , the exact mechanisms by which hyperoxia activates the Nlrp3 inflammasome are currently unknown. However, endogenous danger signals, acting through TLRs, are most likely responsible for the initiation of this innate immune response. We have recently shown that oxidant exposure of high-molecular weight hyaluronan (HMW HA) to oxidant stress results in the formation of low-molecular weight (LMW) HA, and that LMW HA treatment of macrophages results in the production of IL1β (ref. 39 ). Further examination of the mechanisms by which LMW HA is generated and activates the Nlrp3 inflammasome is ongoing. Recombinant, non-glycosylated human IL1ra is currently in clinical use in infants with NOMID. IL1ra treatment of these patients controls the relapsing inflammation and even limits magnetic resonance imaging-identified white matter changes in the brain associated with the inflammatory conditions [40] , [41] . Recent solution of the crystal structure reveals the molecular interactions that allow a greater binding affinity of IL1ra than IL1β itself to the IL1 receptor, thereby resulting in an effective competitive blockade [42] . In a neonatal mouse model of in utero lipopolysaccharide exposure and postnatal hyperoxia exposure, IL1ra treatment was associated with less inflammation and improved alveolarization [43] . These studies confirm the importance of IL1β in the BPD phenotype, but do not address the role of the NLRP3 inflammasome. Importantly, exposure to in utero infection would be a contraindication to the blockade of IL1β, since an inflammatory response is necessary to combat infection. Our studies build on these findings by defining the upstream events in the pathway, by examining the preterm baboon model of BPD that more closely resembles the human condition, and most importantly, definitively implicate the NLRP3 inflammasome in the development of death or BPD in preterm infants. Numerous clinical studies have attempted to develop predictive models for BPD [14] . Of the two best studies, clinical parameters, in particular mechanical ventilator support, were associated with death or BPD at 36 weeks PMA. Ambalavanan et al. [31] , in a study of serum cytokines measured from bloodspots obtained from over 1,000 babies, showed a modest, but significant association between IL1β in the first 3 days of life with death or BPD at 36 weeks PMA. Their study, however, did not examine the lung content of IL1β. The current study suggests that, for infants born at <27 weeks gestation, the lung IL1β parameters are associated with adverse outcome and that, using probability modelling, they are better than gestational age in the prediction of BPD. These data will need to be further validated in a larger cohort of preterm infants. Nevertheless, the data define the population at highest risk by day 3 of life, a time by which infection can be ruled out. Furthermore, since macrophage influx occurs between 7 and 10 days of life, a short-term measure of the effectiveness of potential treatments is provided. We are now poised to conduct pharmacokinetic and safety studies in the baboon model of BPD, followed by studies in human preterm infants to first validate the biomarker findings of this study, and then to develop a randomized controlled trial of either NLRP3 inflammasome or IL1 receptor blockade to potentially decrease the incidence and severity of BPD. Mice Mice with targeted deletion of Nlrp3 ( Nlrp3 −/− ) on a C57/Bl6 background were the kind gift of Vishva Dixit, Ph.D., Genentech, San Francisco, CA. These mice have been characterized previously [11] . Neonatal mouse model of BPD The Animal Care and Use Committee at University of Texas Southwestern Medical Center approved all mouse protocols, which were conducted according to NIH guidelines. Animals were maintained in a barrier condition facility in the Animal Resource Center at UT Southwestern. An established neonatal mouse model of BPD was used with minor modifications [44] , [45] . Newborn mice were used in all studies and litter sizes for each experiment were adjusted to 6–8 pups per treatment group to minimize the effects of differences in nutrition on lung development. All experiments included 6–8 mice per group and all experiments were repeated at least three times. WT or Nlrp3 −/− mice were maintained in either 21% or an 85% O 2 continuously from PN3 to PN14. Oxygen concentration was controlled using the Biospherix controlled atmosphere animal chamber and ProOx monitor (Biospherix Ltd., Rockfield, NY). Nursing mothers were rotated between room air and oxygen-exposed litters daily so as to prevent oxygen toxicity. Both male and female mice were used and animals were killed on PN5, PN10 and PN15 for studies examining time course changes for IL1β, IL1ra and inflammatory cell enzyme activities. All other measurements were made at PN15. In separate treatment studies, newborn WT litters kept in either 21% or 85% O 2 were treated with recombinant IL1ra (Anakinra, Amgen Manufacturing Ltd., Thousand Oaks, CA) at 1 mg kg −1 body weight in 2 μl vehicle (0.7 mg polysorbate 80; 1.29 mg sodium citrate; 5.48 mg sodium chloride and 0.12 mg disodium EDTA in 0.67 ml of sterile water) or vehicle alone via subcutaneous injection every other day from PN3–14. Animals were studied at PN15. In treatment studies to block the formation of the Nlrp3 inflammasome, newborn WT litters kept in 21% or 85% O 2 were treated with 5 μM glyburide, 5 μM glipizide or vehicle (sterile saline) alone. Animals were studied at PN15. The doses of IL1ra and glyburide used were based on published literature in mouse models and in clinical treatment of patients [11] , [41] . Mouse lung harvest Anaesthesia for all studies was attained using an intraperitoneal injection of a Ketamine/Xylazine (87:13 μg kg −1 ) cocktail. BAL was obtained (36 ml kg −1 , total lung capacity) and immediately centrifuged at 500 g for 10 min to isolate cells. Approximately 80% of lavage was routinely recovered. The cellular pellet and the supernatant were separated and frozen at −80 °C until further analysis. The pulmonary artery was perfused with PBS to remove all blood from the lungs. The left lung was inflated to 25 cm H 2 O with 4% paraformaldehyde and placed in 10% neutral formalin for full fixation before processing for paraffin sectioning. The three lobes of the right lung were immediately frozen in liquid nitrogen and stored at −80 °C. Inflation fixed lungs were then processed to obtain 5 μm thick paraffin sections. For each time point, sections were stained with hematoxylin and eosin to examine lung architectural differences using light microscopy. Lung morphometry Alveolarization was determined using RAC. Six random (1,280 × 1,040 pixels) images per section were acquired with a Nikon Eclipse TE300 inverted microscope and Hammamatsu C4742 digital camera, using Metamorph software (Universal Imaging, Westchester, PA). To prevent inadvertent observer bias, an investigator blinded to the assigned groups performed image acquisition and analyses. For each of six images, a perpendicular line was drawn from the centre of a bronchial or bronchiolar airway to either the edge of the lung or the nearest connective tissue septum or airway. A minimum of 40 lines was drawn for each lung, and the number of septae intersected was counted for each line. RAC is a well-established method to quantify alveolarization and previous investigators have confirmed that 40 measurements per lung are sufficient to establish a reliable morphometric assessment of alveolarization [46] , [47] . All RAC calculations were performed using images at × 400 magnification. Isolation of lung cells and flow cytometry Mice were sacrificed on PN15 and perfused lungs were digested in RPMI medium containing collagenase XI (Sigma) and type IV bovine pancreatic DNase (Sigma) to obtain single-cell suspensions. Lung tissues from two mice were pooled to obtain enough cells. After treatment with RBC lysis buffer, single-cell suspensions were surface stained with the following antibodies (eBioscience): CD45 (clone 30-F11, PE-Cy7, 1:400 dilution), Ly6G (clone 1A8, FITC, 1:200 dilution), F4/80 (clone BM8, APC, 1:400 dilution), CD4 (Per-CP Cy5.5, 1:400 dilution), CD11c (clone HL3, APC Cy-7, 1:400 dilution) and CD86 (clone GL3, PE, 1:400 dilution). Flow cytometry was performed using BD FACS Canto cytometer (BD Bioscience) at the University of Texas Southwestern Flow Cytometry Core Facility, and data were analysed with FlowJo software (TreeStar, Ashland, OR). Isolation of alveolar and BMDMs Alveolar macrophages were isolated by BAL of adult mice. After appropriate anaesthesia, the trachea on the ventral side of the neck was exposed and a 20-G intramedic adaptor (Becton Dickinson, Sparks, MD) was inserted and attached to a 1-ml syringe. BAL was accomplished using sterile, ice-cold normal saline with 0.6 mM EDTA in aliquots of 1 ml to a total volume of 10 ml. The lavage fluid was centrifuged at 300 g for 10 min to pellet alveolar macrophages. The pelleted cells were resuspended and cultured in a 12-well culture plate at 37 °C with 5% CO 2 at a concentration of 3 × 10 5 cells per well in 1 ml RPMI 1640 medium (Sigma Chemical Co., St Louis, MO) with heat inactivated 10% fetal bovine serum and 1% penicillin and streptomycin. BMDMs were obtained from the same mice. Briefly, bone marrow was flushed from the tibia and femur of each mouse with macrophage medium (RPMI with 10% FCS, 20% L929 conditioned medium, 1% penicillin/streptomycin/glutamine) under sterile conditions. Marrow cells were made into a single-cell suspension by gentle pipetting and straining. Cells were centrifuged and resuspended, red blood cells were lysed by exposure to RBC lysis buffer, and then cells were cultured in macrophage medium. Non-adherent cells were replated and provided fresh medium. Cells were allowed to further differentiate for 3 days and were then used for assays. Alveolar and BMDM were either maintained quiescent or treated with either lipopolysaccharide (1 μg ml −1 , Sigma) to stimulate TLR4, or the endotoxin-free, synthetic TLR2 ligand, tripalmitoyl-S-glycero-Cys-(Lys)4 (5 μM, Invivogen, San Diego, CA) for 16 h. NAG activity was determined as described below. Non-human primate model of BPD All animal procedures were reviewed and approved by the Animal Care and Use Committees of the Southwest Foundation for Biomedical Research and the University of Texas Southwestern Medical Centre. The Southwest Foundation for Biomedical Research (San Antonio, TX) provided frozen baboon lung tissue and BAL samples. Gestational age controls and samples to determine ontogeny were obtained by caesarian section at 125, 140, 160, 175 days gestation and at 185 days with the onset of labour. For the BPD model, premature baboons that were delivered by hysterotomy at 125 days were intubated, treated with exogenous surfactant (Survanta; donated by Ross Laboratories, Columbus, OH) and maintained on pressure-limited, time-cycled infant ventilators (donated by Infant Star; Infrasonics, San Diego, CA) for 2, 6, or 14 days. The ventilator settings were adjusted to maintain the arterial carbon dioxide tension (PaCO 2 ) between 45 and 55 mm Hg and oxygen was provided on a PRN basis to maintain the arterial oxygen tension (PaO 2 ) between 55 and 70 mm Hg. Animals that were killed at 14 days had pathologic and biochemical findings that were characteristic of the new BPD seen in human infants as described previously [48] , [49] , [50] . Baboons that were delivered at 125 days or 140 days and killed immediately, served as the gestational controls. Lung tissue was used to determine the mRNA content of IL1β, caspase-1 activity and p20-active caspase-1 immunoblot. Tracheal aspirates and BAL were used to determine protein contents of IL1β, IL1ra and SCIgA. Preterm neonates with respiratory failure The Institutional Review Board of The University of Texas Southwestern Medical Center approved the human subject protocol and granted waiver of consent status as samples were obtained from routine clinical care and were handled in a completely de-identified manner. We conducted a prospective cohort study of preterm neonates at risk of developing BPD. Infants born between 24 0/7 and 31 6/7 weeks gestational age, and who were intubated for respiratory failure were included in the study. Infants with proven sepsis (as evidenced by a positive blood culture), perinatal asphyxia, major congenital anomalies and those provided comfort care only, were excluded from the study. BPD was diagnosed using the NIH physiologic definition using a room air challenge test performed at 36 weeks PMA [51] . Because death is a competing outcome for BPD, adverse outcome was defined as death or BPD at 36 weeks PMA and was used as the primary outcome for this study. Tracheal aspirates, obtained as a part of routine care, were collected daily for the first 10 days of life, and then every 7–10 days thereafter until the infant was extubated. Samples were immediately spun at low speed (500 g ) to separate the cell pellet from supernatant and each was frozen at −80 °C until further analyses. Each of the samples was labelled by a unique study number. Investigators participating in biomarker measurements were blinded to patient characteristics and outcomes. The contents of IL1β, IL1ra and SCIgA were measured in BAL supernatant, whereas MPO and NAG activities (see below) were determined in the cell pellets obtained by BAL. Antibodies The following antibodies were used in either immunostaining or immunoblot studies. Anti-caspase-1 (Cat.# 06-503, Millipore, Temecula, CA, 1:1,000 dilution); Anti β-actin (Cat.# 4967, Cell Signaling, Boston, MA, 1:1,000 dilution); Anti-YM1 (Cat.# 01404, StemCell Technologies, Vancouver, Canada, 1:100 dilution); Anti-CD11c (Cat.# ab11029, Abcam, Cambridge, MA, 1:100 dilution). RNA isolation and quantitative real-time PCR Total RNA was extracted from lung tissues using RNeasy Plus Mini Kit (QIAGEN Inc., Valencia, CA), following the manufacturer’s instructions. Extracted RNA concentration of each sample was quantified using a NanoDrop ND-1000 Spectrophotometer (Thermo Fisher Scientific, Wilmington, DE). Reverse transcription was performed with 1 μg of total RNA in a 20 μl volume using iScript cDNA synthesis kit (Bio-Rad, Hercules, CA). The real-time quantitative PCR were performed on a 7900 HT fast real-time PCR system (Applied Biosystems, Foster, CA) using 2 μl cDNA, 7 μl diethylpyrocarbonate water, 10 μl SsoFast Probes Supermix with ROX (Bio-Rad, Hercules, CA) and 1 μl primer of TaqMan Gene Expression Assay. Forty cycles of amplification were performed. Cycle threshold (Ct) values were determined using SDS2.4 software. The gene of interest was normalized to the Ct value of the endogenous reference gene, 18 s rRNA, using the ΔCt method described by Pfaffl [52] . TaqMan gene expression assays (Applied Biosystems) were used for each gene as pre-made primers/probe sets. The assay IDs are mouse Mm01336189_m1 (IL1β), Mm00434225_m1 (IL18), Mm00446186_m1 (IL1ra), Mm00440502_m1 (iNOS), Human Hs00174097_m1 (IL1β), Hs00893626_m1 (IL1RA), Hs99999901_s1 (18 s rRNA). Multiplex cytokine array and ELISAs BAL from two mice per group was pooled resulting in three samples per group per experiment. BAL (50 μl) was used in the Discovery Mouse Cytokine/Chemokine 31-Plex Array (Eve Technologies, Calgary, Alberta, Canada). Mouse and human IL1β, IL1ra, IL18, TGFβ1 and TNFα were also analysed in BAL or lung homogenates with commercially available ELISA kits (R&D systems, Minneapolis, MN) according to the manufacturer’s instructions. Human SCIgA was measured in BAL from non-human primate and human samples using Secretory IgA ELISA kit (Eagle Biosciences, Nashua, NH). There was insufficient BAL from mouse studies to measure SCIgA in addition to IL1β and IL1ra. Caspase-1 activity assay Caspase-1 activity was analysed using WEHD-AFC substrate and a caspase-1 fluorometric assay kit as per manufacturer’s instructions (Cat. #BF12100, R&D Systems). Western blot analysis Western blot analysis was performed using the NOVEX NuPAGE electrophoresis system (Invitrogen, Grand Island, NY) with 1.5 mm 4–12% Bis–Tris gels according to manufacturer's instructions. Briefly, 25 μg of lung homogeneous was loaded to each well and gels were run at 100 V at 4 °C for 2 h in NuPAGE MOPS SDS running buffer under reducing conditions. Proteins were transferred to nitrocellulose membrane at 80 V for 60 min at 4 °C. The membrane was then blocked for 1 h at room temperature with 5% BSA in Tween/Tris buffered saline (TTBS; 100 mM Tris base, 1.5 M NaCl adjusted to pH 7.4 with 0.1% Tween 20). Immunoblots were then incubated with caspase-1 antibody (1:1,000, Millipore, Temecula, CA) overnight at 4 °C. The following day, the membrane was washed with TTBS three times, for 20 min each time. A horseradish peroxidase-conjugated goat anti-rabbit antibody (1:10,000, Santa Cruz Biotechnology, Santa Cruz, CA), used as the secondary antibody, was applied for 1 h at room temperature. Following this, the membrane was washed with TTBS followed by two 10-min washes with TBS. The blots were developed using a chemiluminescence system (Amersham Pharmacia Biotech, Piscataway, NJ). Complete western blots without cropping are shown in Supplementary Fig. 5 . MPO and NAG activity assays The contents of neutrophils and macrophages in cell pellets obtained by BAL were measured on PN5, 10 and 15 by assaying MPO and NAG activities, respectively, as previously described [39] . Briefly, the cell pellet from each mouse was lysed with 50 μl RIPA buffer (Sigma, St Louis, MO). For MPO activity, 25 μl of cell lysate or 4.15–83 mU of MPO standards (Sigma, St Louis, MO) were loaded in 96-well plates. Sixty microliters of 0.1 M K 2 PO 4 , 20 μl of 0.5% H 2 O 2 and 20 μl of 1.25 mg ml −1 O-diansidine (ICN Biomedicals, Irvine, CA) were added to each well. After incubation at room temperature for 15 min, the reaction was stopped by the addition of 20 μl 1% sodium azide. The change in absorbance at 450 nm over the 15 min provided an index of MPO activity and correlates with neutrophil content. For NAG activity, 20 μl of cell lysate or 25–400 μU of β-Nacetylglucosaminidase standard (Sigma, St Louis, MO) was loaded in 96-well plates. Ten microliters of 0.1% Triton × and 20 μl of 15 mM p -nitrophenyl N-acetyl-β- D -glucosaminide (Sigma, St Louis, MO) were added to each well. After incubation at 37 °C for 30 min, 200 μl of 0.2 M sodium carbonate was added to each well to stop the reaction. The change in absorbance at 405 nm was measured as an index of NAG activity and correlates with macrophage content. Final results were obtained by multiplying MPO values by 2 and NAG values by 2.5 to account for dilution during the assays. Immunostaining and macrophage phenotyping Macrophage phenotypes were identified and quantified by immunofluorescence staining with specific antibodies, using CD11c (Abcam, Cambridge, MA, 1:100 dilution) for M1, classically activated macrophages and YM1 (StemCell Technologies, Vancouver, Canada, 1:100 dilution) for M2, alternatively activated macrophages. After paraffin removal and rehydration, endogenous fluorescence was blocked with 0.1% sodium borohydride for 10 min followed by incubation with fresh 1 M glycine in PBS for 30 min. Nonspecific binding was blocked by incubation with 100% goat serum for overnight at 4 °C. Sections were incubated with rabbit anti-mouse YM1 or CD11C overnight at 4 °C. After washing, the slides were incubated with goat anti-rabbit FITC-conjugated secondary antibody (1:500 dilution) for 60 min. Slides were washed and mounted with Fluoromount-G (Southern Biotechnology Associates, Birmingham, AL). Two independent and blinded observers counted the absolute number of YM1- or CD11c- positive cells as well as a per cent of total cells per high power field to quantify macrophage accumulation in at least three animals from each group. Each observer selected five random fields from different portions of the lung in one slide section for counting and used sections obtained from different areas of lung tissue to ensure adequate sampling. In addition, all sections were observed under low-power magnification to ensure that all areas of the lung section had been included in the determinations. Terminal transferase dUTP nick-end labelling In situ TUNEL for the detection of apoptotic was performed on PN15 tissue sections using an in situ cell death detection fluorescence kit (Roche Diagnostics GmbH, Mannheim, Germany) as per manufacturer’s instructions. TUNEL-positive cells were counted in at least 10 non-overlapping HPFs (× 400 magnification) from three to four animals per group. Statistical analyses To determine group sizes necessary for adequate statistical power, power analysis was performed using preliminary data sets of IL1β concentrations in the BAL from mice. Group sample sizes of 6 in each group were predicted to achieve 95% power to detect a difference of 60 between the null hypothesis that both group means were 11.44 and the alternative hypothesis that the mean of group 2 is 71.7 with estimated group s.d. of 1.98 and 32.3 and with a significance level (alpha) of 0.05 using a two-sided two-sample t -test. The investigators were blinded to group allocation during collection and analysis of the data, and all inclusion/exclusion criteria were pre-established. Data are expressed as mean±s.e.m. Normally distributed variables were analysed by analysis of variance or unpaired Student’s t -test. Non-parametric variables were compared using Mann–Whitney rank-sum tests. Biomarker data were log-transformed to achieve a normal distribution and plotted as box and whisker plots where the boxes represent 25th and 75th percentiles, the bars within the boxes are the medians, and error bars represent one s.d. from the mean. Results were analysed in epochs consisting of days 1–3, 4–6 and 7–10 for samples obtained daily. Since gestational age is a known confounder for the development of BPD, correlations between gestational age and biomarkers were examined. All statistical analyses were conducted using GraphPad Prism 6 software (GraphPad Software Inc., San Diego, CA). Logistic regression was performed with SPSS software (IBM SPSS version 19) to control for the contribution of gestational age to the content of each biomarker. Using mixed model methodology, probability analysis was performed to compare the predictive ability of biomarkers combined with gestational age with gestational age alone. Significance for all statistical tests is shown in the figures and P <0.05 was considered significant. How to cite this article: Liao, J. et al. The NLRP3 inflammasome is critically involved in the development of bronchopulmonary dysplasia. Nat. Commun. 6:8977 doi: 10.1038/ncomms9977 (2015).